Oestrogen sulfotransferase ablation sensitizes mice to sepsis Sepsis is the host’s deleterious systemic inflammatory response to microbial infections. Here we report an essential role for the oestrogen sulfotransferase (EST or SULT1E1), a conjugating enzyme that sulfonates and deactivates estrogens, in sepsis response. Both the caecal ligation and puncture (CLP) and lipopolysaccharide models of sepsis induce the expression of EST and compromise the activity of oestrogen, an anti-inflammatory hormone. Surprisingly, EST ablation sensitizes mice to sepsis-induced death. Mechanistically, EST ablation attenuates sepsis-induced inflammatory responses due to compromised oestrogen deactivation, leading to increased sepsis lethality. In contrast, transgenic overexpression of EST promotes oestrogen deactivation and sensitizes mice to CLP-induced inflammatory response. The induction of EST by sepsis is NF-κB dependent and EST is a NF-κB-target gene. The reciprocal regulation of inflammation and EST may represent a yet-to-be-explored mechanism of endocrine regulation of inflammation, which has an impact on the clinical outcome of sepsis. Sepsis, the leading cause of death in the intensive care unit, is the host’s deleterious systemic inflammatory response to microbial infections. The caecal ligation and puncture (CLP) and treatment with lipopolysaccharide (LPS) are two commonly used sepsis models. In the CLP model, sepsis originates from a polymicrobial infection within the abdominal cavity [1] . Toll-like receptor 4 (TLR4) has been reported to contribute to bacterial clearance and the host inflammatory response in sepsis [2] . The bacterial LPS elicits its inflammatory actions through the TLR4, which will lead to the activation of nuclear factor-κB (NF-κB), a transcriptional factor that regulates a battery of inflammatory genes [2] . The oestrogen sulfotransferase (EST or SULT1E1) is a cytosolic sulfotransferase best known for its activity in sulfonating and deactivating oestrogen, an anti-inflammatory hormone. This is because the sulfonated estrogens cannot bind to and activate the oestrogen receptor [3] . Consistent with the role of EST in oestrogen deactivation, EST ablation in mice resulted in structural and functional lesions in the testis [4] and placenta [5] . The basal expression of hepatic EST is low, but its expression is highly inducible in response to ligands for several nuclear receptors [6] , [7] , [8] and insulin resistance/type 2 diabetes [9] , [10] . The expression of many drug-metabolizing enzymes is suppressed by inflammation [11] . It is unclear whether and how EST is regulated by sepsis, and if so, whether this regulation can impact oestrogen homeostasis and sepsis response. The anti-inflammatory activities of estrogens have long been recognized, but not without controversies including in the context of endotoxaemia. For example, estrogens or oestrogen receptor agonists have been reported to increase serum tumour necrosis factor (TNF) levels and mortality in endotoxaemic mice [12] , [13] , [14] , [15] . Having known that EST is a key enzyme in the metabolic deactivation of estrogens, it is unclear whether the hepatic expression and regulation of EST affect the host’s response to sepsis. Here we report that EST is markedly induced by sepsis in a NF-κB-dependent manner. EST plays an important role in sepsis response in that EST ablation attenuates sepsis-induced inflammatory responses and sensitizes mice to sepsis-induced lethality. Sepsis induced EST expression and deactivated estrogens Knowing the expression of many drug-metabolizing enzymes is suppressed by inflammation [11] , we were surprised to find that the hepatic expression of EST was markedly increased in mice subjected to CLP ( Fig. 1a ) or LPS treatment ( Fig. 1b ) at both the mRNA and protein levels. The higher levels of TNFα and interleukin (IL)-6 in the CLP group ( Fig. 1a ) indicated inflammation and success of the sepsis models. The induction was both liver specific and EST specific, because the expression of EST in the white adipose tissue was not affected ( Fig. 1b ) and the hepatic expression of Cyp3a11, a typical drug-metabolizing enzyme, was decreased in both models ( Fig. 1c ). The induction of EST was also confirmed at the enzymatic level, as shown by increased oestrogen sulfation in the liver cytosols isolated from CLP- or LPS-treated mice ( Fig. 1d ). At the functional level, treatment of 4-week-old intact virgin female mice with LPS resulted in a significantly reduced circulating oestradiol level ( Fig. 1e ). Treatment of female mice with LPS also increased the urinary output of oestrogen sulfate ( Fig. 1f ). Moreover, both the oestrogen-responsive uterine epithelial proliferation ( Fig. 1g ) and gene expression ( Fig. 1h ) was compromised in LPS-treated mice, and these effects were abolished in EST null (EST−/−) mice [4] . 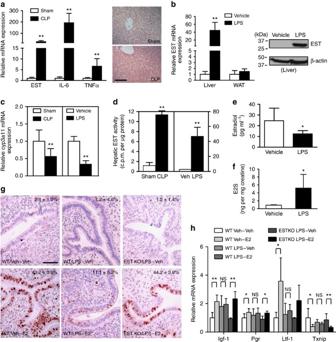Figure 1: Sepsis-induced EST gene expression and compromised oestrogen activity. (a) The mRNA expression of EST, IL-6 and TNFα (left) and immunostaining of EST (right) in the liver of mice 12 h after CLP. (b) The mRNA expression of EST in the liver and white adipose tissue (left) and protein expression of EST (right) 12 h after a single i.p. injection of LPS (5 mg kg−1). The locations of protein size markers in the western blotting are labelled. Hepatic mRNA expression of Cyp3a11 (c) and EST activity (d) of mice described inaandb. (e) Four-week-old virgin female mice treated with LPS were measured for endogenous E2levels. Mice received a single i.p. dose of LPS (5 mg kg−1) 24 h before being killed. (f) Urinary output of oestrogen sulfate in mice treated with vehicle or LPS (1 mg kg−1). (g) BrdU labelling and immunostaining on uterine paraffin sections from mice, indicated genotype and drug treatment. All mice were ovariectomized 7 days before the oestrogen treatment. Mice received a single subcutaneous injection of vehicle or E2(20 μg kg−1) 20 h before being killed. Mice were labelled for BrdU (60 mg kg−1) 2 h before being killed. Percentages of BrdU-positive nuclei are quantitated and labelled. When applicable, mice were pretreated with LPS (5 mg kg−1) for 12 h before the E2treatment. The original magnification is × 400 for all panels. KO, knockout. (h) Expression of uterine oestrogen- responsive genes measured by real-time PCR. Igf-1, insulin-like growth factor 1; Ltf, lactoferrin; Pgr, progesterone receptor; Txnip, thioredoxin-interacting protein. The Sham/vehicle (Veh) and the CLP/LPS groups contained four and five independent mice per group, respectively. The mRNA expression levels in the control groups ina–c, andhwere arbitrarily set at 1. Results are presented as means±s.d. *P<0.05; **P<0.01; NS, statistically not significant. Student’st-test was used to calculate thePvalues. Scale bar, 50 μm in the histographs ofaandg. Figure 1: Sepsis-induced EST gene expression and compromised oestrogen activity. ( a ) The mRNA expression of EST, IL-6 and TNFα (left) and immunostaining of EST (right) in the liver of mice 12 h after CLP. ( b ) The mRNA expression of EST in the liver and white adipose tissue (left) and protein expression of EST (right) 12 h after a single i.p. injection of LPS (5 mg kg −1 ). The locations of protein size markers in the western blotting are labelled. Hepatic mRNA expression of Cyp3a11 ( c ) and EST activity ( d ) of mice described in a and b . ( e ) Four-week-old virgin female mice treated with LPS were measured for endogenous E 2 levels. Mice received a single i.p. dose of LPS (5 mg kg −1 ) 24 h before being killed. ( f ) Urinary output of oestrogen sulfate in mice treated with vehicle or LPS (1 mg kg −1 ). ( g ) BrdU labelling and immunostaining on uterine paraffin sections from mice, indicated genotype and drug treatment. All mice were ovariectomized 7 days before the oestrogen treatment. Mice received a single subcutaneous injection of vehicle or E 2 (20 μg kg −1 ) 20 h before being killed. Mice were labelled for BrdU (60 mg kg −1 ) 2 h before being killed. Percentages of BrdU-positive nuclei are quantitated and labelled. When applicable, mice were pretreated with LPS (5 mg kg −1 ) for 12 h before the E 2 treatment. The original magnification is × 400 for all panels. KO, knockout. ( h ) Expression of uterine oestrogen- responsive genes measured by real-time PCR. Igf-1, insulin-like growth factor 1; Ltf, lactoferrin; Pgr, progesterone receptor; Txnip, thioredoxin-interacting protein. The Sham/vehicle (Veh) and the CLP/LPS groups contained four and five independent mice per group, respectively. The mRNA expression levels in the control groups in a – c , and h were arbitrarily set at 1. Results are presented as means±s.d. * P <0.05; ** P <0.01; NS, statistically not significant. Student’s t -test was used to calculate the P values. Scale bar, 50 μm in the histographs of a and g . Full size image Kupffer cells were required for the optimal EST induction We showed that the isolated Kupffer cells expressed EST and treatment of Kupffer cells with LPS induced the expression of EST ( Fig. 2a ). The expression of EST in Kupffer cells was also induced by the treatment of Pam3CSK4, a synthetic triacylated lipopeptide and TLR2 ligand [16] , but not by the treatment of ODN1826, a Class B CpG oligonucleotide, and TLR9 ligand [17] ( Fig. 2a ). The success of the Kupffer cells’ isolation was confirmed by measuring the expression of the macrophage marker gene F4/80 ( Fig. 2b ). In vivo pharmacological depletion of Kupffer cells by treating mice with gadolinium chloride (GdCl 3 ) (ref. 18 ) attenuated but did not abolish the CLP- and LPS-responsive induction of EST ( Fig. 2c ). The sepsis-responsive increase of hepatic IL-6 mRNA expression ( Fig. 2c ) and serum level of IL-6 ( Fig. 2d ) were also attenuated in GdCl 3 -treated mice. The efficiency of Kupffer cell depletion was confirmed by the decreased hepatic expression of F4/80 ( Fig. 2e ). These results suggested that both the hepatocytes and Kupffer cells contribute to the basal and sepsis-inducible expression of EST in the liver. 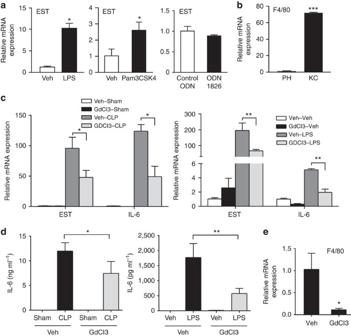Figure 2: Kupffer cells were required for the optimal induction of EST by sepsis. (a) The expression of EST in primary Kupffer cells treated with vehicle (Veh) or LPS (1 μg ml−1, left panel), lipopeptide Pam3CSK4 (300 ng ml−1, middle panel) or CpG oligonucleotide ODN1826 (10 μg ml−1, right panel). (b) The quality of the Kupffer cell isolation was confirmed by comparing the expression of the macrophage marker geneF4/80in primary hepatocytes (PH) and Kupffer cells (KC). (c) Mice pretreated with vehicle or GdCl3were subjected to CLP or LPS (5 mg kg−1) treatment. Mice were killed 12 h after CLP or LPS treatment and measured for EST and IL-6 mRNA expression. (d) Serum level of IL-6 in mice subjected to CLP or LPS treatment. (e) The efficiency of GdCl3-induced Kupffer cell depletion was confirmed by the measurement of F4/80 expression. The Kupffer cells inaandbwere pooled from two mice and results were obtained from triplicate assay. The Sham/Vehicle and the CLP/LPS groups inc–econtained four and five independent mice per group, respectively. The mRNA expression levels in the control groups ina–c, andewere arbitrarily set at 1. Results are presented as means±s.d. *P<0.05; **P<0.01; ***P<0.001. Student’st-test was used to calculate thePvalues. Figure 2: Kupffer cells were required for the optimal induction of EST by sepsis. ( a ) The expression of EST in primary Kupffer cells treated with vehicle (Veh) or LPS (1 μg ml −1 , left panel), lipopeptide Pam3CSK4 (300 ng ml −1 , middle panel) or CpG oligonucleotide ODN1826 (10 μg ml −1 , right panel). ( b ) The quality of the Kupffer cell isolation was confirmed by comparing the expression of the macrophage marker gene F4/80 in primary hepatocytes (PH) and Kupffer cells (KC). ( c ) Mice pretreated with vehicle or GdCl 3 were subjected to CLP or LPS (5 mg kg −1 ) treatment. Mice were killed 12 h after CLP or LPS treatment and measured for EST and IL-6 mRNA expression. ( d ) Serum level of IL-6 in mice subjected to CLP or LPS treatment. ( e ) The efficiency of GdCl 3 -induced Kupffer cell depletion was confirmed by the measurement of F4/80 expression. The Kupffer cells in a and b were pooled from two mice and results were obtained from triplicate assay. The Sham/Vehicle and the CLP/LPS groups in c – e contained four and five independent mice per group, respectively. The mRNA expression levels in the control groups in a – c , and e were arbitrarily set at 1. Results are presented as means±s.d. * P <0.05; ** P <0.01; *** P <0.001. Student’s t -test was used to calculate the P values. Full size image EST is a transcriptional target of NF-κB The CLP- and LPS-responsive induction of EST was TLR4 dependent, because this induction was decreased in two independent strains of TLR4 mutant mice [19] , [20] ( Supplementary Fig. 1a ). The sepsis-responsive induction of IL-6 gene expression and increased serum level of IL-6 was also attenuated in TLR4 mutant mice ( Supplementary Fig. 1b ). NF-κB is a key inflammatory transcriptional factor downstream of TLR4 (ref. 21 ). A putative NF-κB-binding site was bioinformatically predicted in the mouse EST gene promoter ( Fig. 3a ), and its binding to p65, a major subunit of NF-κB, was confirmed by electrophoretic mobility shift assay (EMSA) ( Fig. 3a ). A luciferase reporter gene that contained 2.5 kb of the EST gene promoter, but not its variants with the EST/κB site mutated or deleted, was activated by the co-transfection of p65 in HepG2 cells ( Fig. 3b ). The HepG2 cells contained the machinery for the p65 responses, because transfection of p65 induced the expression of pro-inflammatory genes IL-6 and MCP-1 in these cells ( Supplementary Fig. 2 ). The recruitment of p65 onto the EST gene promoter in vivo was confirmed by chromatin immunoprecipitation (ChIP) assay on the liver of LPS-treated mice ( Fig. 3c ). We also showed that treatment with pyrrolidine dithiocarbamate (PDTC), a pharmacological inhibitor of NF-κB [22] , attenuated CLP- and LPS-responsive induction of EST ( Fig. 3d ). These results demonstrated that EST is a transcriptional target of NF-κB. 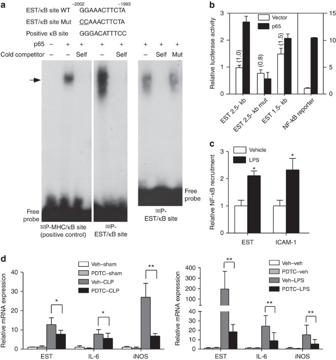Figure 3: EST is a transcriptional target of NF-κB and pharmacological inhibition of NF-κB attenuated the sepsis-responsive induction of EST. (a) Top: The sequences of mouse EST NF-κB responsive elements and its mutant (Mut) variant. The mutated nucleotides are underlined. The sequence of the positive control κB site derived from the major histocompatibility complex (MHC) class II-associated invariant chain gene is also shown. Bottom: The binding of p65 protein to the EST NF-κB site was shown by EMSA. (b) Activation of the mouse EST promoter reporter genes or their mutant variants by the co-transfection of p65. HepG2 cells were co-transfected with indicated reporters and vectors. Transfected cells were cultured for 24 h before luciferase assay. The luciferase activity was normalized to the β-gal activity from the co-transfected β-gal expression vector. All EST promoter activities were normalized to EST 2.5-kb vector, which was arbitrarily set at 1. The relative basal activities of the WT and mutant EST promoters are labelled. The NF-κB reporter gene was included as the positive control. (c) ChIP assays to show the recruitment of p65 onto the EST gene promoter. Eight-week-old WT female mice were injected with a single dose of vehicle (Veh; saline) or LPS (5 mg kg−1) 12 h before being killed. The DNA precipitates were analysed by real-time PCR. The recruitment of p65 to the ICAM-1 gene promoter was included as a positive control. The recruitment of p65 in the vehicle group was arbitrarily set at 1. (d) Pharmacological inhibition of NF-κB attenuated the LPS- and CLP-responsive induction of EST. WT female mice were treated with a single i.p. dose of PDTC (200 mg kg−1) 1 h before they were challenged with LPS (5 mg kg−1) or subjected to CLP. The mice were killed 12 h after LPS or CLP and measured for the mRNA expression of EST, IL-6 and iNOS. Experiments incanddcontained five independent mice per group. The mRNA expression levels in the control groups indwere arbitrarily set at 1. Results are presented as means±s.d. *P<0.05; **P<0.01. Student’st-test was used to calculate thePvalues. Figure 3: EST is a transcriptional target of NF-κB and pharmacological inhibition of NF-κB attenuated the sepsis-responsive induction of EST. ( a ) Top: The sequences of mouse EST NF-κB responsive elements and its mutant (Mut) variant. The mutated nucleotides are underlined. The sequence of the positive control κB site derived from the major histocompatibility complex (MHC) class II-associated invariant chain gene is also shown. Bottom: The binding of p65 protein to the EST NF-κB site was shown by EMSA. ( b ) Activation of the mouse EST promoter reporter genes or their mutant variants by the co-transfection of p65. HepG2 cells were co-transfected with indicated reporters and vectors. Transfected cells were cultured for 24 h before luciferase assay. The luciferase activity was normalized to the β-gal activity from the co-transfected β-gal expression vector. All EST promoter activities were normalized to EST 2.5-kb vector, which was arbitrarily set at 1. The relative basal activities of the WT and mutant EST promoters are labelled. The NF-κB reporter gene was included as the positive control. ( c ) ChIP assays to show the recruitment of p65 onto the EST gene promoter. Eight-week-old WT female mice were injected with a single dose of vehicle (Veh; saline) or LPS (5 mg kg −1 ) 12 h before being killed. The DNA precipitates were analysed by real-time PCR. The recruitment of p65 to the ICAM-1 gene promoter was included as a positive control. The recruitment of p65 in the vehicle group was arbitrarily set at 1. ( d ) Pharmacological inhibition of NF-κB attenuated the LPS- and CLP-responsive induction of EST. WT female mice were treated with a single i.p. dose of PDTC (200 mg kg −1 ) 1 h before they were challenged with LPS (5 mg kg −1 ) or subjected to CLP. The mice were killed 12 h after LPS or CLP and measured for the mRNA expression of EST, IL-6 and iNOS. Experiments in c and d contained five independent mice per group. The mRNA expression levels in the control groups in d were arbitrarily set at 1. Results are presented as means±s.d. * P <0.05; ** P <0.01. Student’s t -test was used to calculate the P values. Full size image EST ablation sensitized mice to sepsis-induced death Knowing oestrogen is an anti-inflammatory hormone, we were surprised to find that EST ablation markedly sensitized female mice to CLP-induced death ( Fig. 4a ). This sensitizing effect of EST ablation was completely abolished on ovariectomy ( Fig. 4a ), suggesting this effect was oestrogen dependent. The EST null phenotype was recapitulated in wild-type (WT) mice pretreated with triclosan (5-chloro-2(2,4-dichlorophenoxy)-phenol), a pharmacological inhibitor of EST [23] , [24] . Since an efficient inflammatory response is a key survival response to release pro-inflammatory cytokines and chemokines [25] , we reasoned that EST ablation may have attenuated CLP- and LPS-responsive inflammatory response and thus sensitized mice to sepsis-induced death. Indeed, the CLP- and LPS-responsive induction of IL-6 and IL-1β/TNFα mRNA expression was attenuated in EST−/− mice compared with their WT counterparts ( Fig. 4b ). The serum levels of IL-6 and TNFα in the CLP-treated EST−/− mice and LPS-treated EST−/− mice were also lower ( Fig. 4c ). The suppression of oestrogen-responsive genes observed in the liver of CLP- and LPS-treated WT mice was abolished in EST−/− mice ( Fig. 4d ), consistent with the loss of EST-mediated oestrogen deprivation. The expression of macrophage marker genes Cd68 and F4/80 was indistinguishable between the WT and EST−/− mice, suggesting that the EST ablation alone had little effect on the numbers of macrophages/Kupffer cells and expression of inflammatory marker genes ( Supplementary Fig. 3 ). CLP is known to cause histological damages to the liver, lung [26] , heart [27] and kidney [28] . We found the liver ( Fig. 4e ), heart ( Supplementary Fig. 4a ) and kidney ( Supplementary Fig. 4b ) histology was not different between the WT and EST−/− mice. In contrast, the lung of the EST−/− mice exhibited much more pronounced interstitial oedema ( Fig. 4e ). Although the mechanism remains to be defined, these results suggested that the heightened lung injury might have contributed to the worsened survival of the EST−/− mice in response to CLP. In the CLP model, the bacterial count in the peritoneal fluid was not significantly different between the WT and EST−/− mice ( Fig. 4f ). The male EST−/− also exhibited heightened sensitivity to CLP-induced death ( Fig. 4g ). 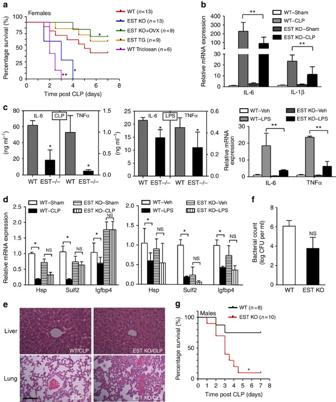Figure 4: EST ablation sensitized mice to sepsis-induced death. (a) Seven-day CLP survival in female mice of indicated genotypes and treatment. OVX, ovariectomy. When necessary, CLP was performed 7 days after ovariectomy. Also when necessary, mice were given daily subcutaneous injections of triclosan (10 mg kg−1) beginning 3 days before CLP. *P<0.05, compared with the WT group. (b) CLP- and LPS-responsive expression of inflammatory cytokines in female WT and EST−/− mice 12 h after CLP or a single i.p. injection of LPS (5 mg kg−1). (c) Serum IL-6 and TNFα levels in mice subjected to CLP or LPS treatment. (d) The hepatic expression of oestrogen-responsive genes in mice subjected to CLP or LPS treatment. The liver and lung histology (e, scale bar, 50 μm) and the bacterial count in the peritoneal fluid (f) of female WT and EST−/− mice 16 h after CLP. (g) Seven-day CLP survival in male WT and EST−/− mice. The animal numbers inaandgare labelled. Experiments inb–fcontained five independent mice per group. The mRNA expression levels in the control groups inbanddwere arbitrarily set at 1. Results are presented as means±s.d. *P<0.05, compared with the WT group. Log-rank (Mantel–Cox) test was used to calculate thePvalues inaandg. Student’st-test was used to calculate thePvalues inb–d,andf. CFU, colony-forming unit; Veh, vehicle. Figure 4: EST ablation sensitized mice to sepsis-induced death. ( a ) Seven-day CLP survival in female mice of indicated genotypes and treatment. OVX, ovariectomy. When necessary, CLP was performed 7 days after ovariectomy. Also when necessary, mice were given daily subcutaneous injections of triclosan (10 mg kg −1 ) beginning 3 days before CLP. * P <0.05, compared with the WT group. ( b ) CLP- and LPS-responsive expression of inflammatory cytokines in female WT and EST−/− mice 12 h after CLP or a single i.p. injection of LPS (5 mg kg −1 ). ( c ) Serum IL-6 and TNFα levels in mice subjected to CLP or LPS treatment. ( d ) The hepatic expression of oestrogen-responsive genes in mice subjected to CLP or LPS treatment. The liver and lung histology ( e , scale bar, 50 μm) and the bacterial count in the peritoneal fluid ( f ) of female WT and EST−/− mice 16 h after CLP. ( g ) Seven-day CLP survival in male WT and EST−/− mice. The animal numbers in a and g are labelled. Experiments in b – f contained five independent mice per group. The mRNA expression levels in the control groups in b and d were arbitrarily set at 1. Results are presented as means±s.d. * P <0.05, compared with the WT group. Log-rank (Mantel–Cox) test was used to calculate the P values in a and g . Student’s t -test was used to calculate the P values in b – d ,and f . CFU, colony-forming unit; Veh, vehicle. Full size image Overexpression of EST sensitized mice to sepsis inflammation In a gain of function model, we created transgenic mice overexpressing EST in the liver/hepatocytes by using the ‘Tet-Off’ transgenic (TG) system and the hepatocyte-specific liver-enriched activator protein (Lap) gene promoter as outlined in Fig. 5a . The liver-specific overexpression of EST was confirmed by real-time PCR ( Fig. 5b ). The expression of EST in the lymphoid organ spleen was indistinguishable between the WT and TG mice ( Fig. 5b ). As shown in Fig. 5c , the hepatic levels of E 1 and E 2 were significantly lower in TG mice. Moreover, both the oestrogen-responsive uterine epithelial proliferation ( Fig. 5d ) and gene expression ( Fig. 5e ) were attenuated in TG mice. When challenged with CLP or LPS, the TG mice showed more profound induction of pro-inflammatory cytokines ( Fig. 5f ). The serum level of IL-6 in CLP- or LPS-treated TG mice was also higher than their WT counterparts ( Fig. 5g ). The TG mice also showed a modestly improved survival to CLP ( Fig. 4a ), which may have been accounted for by the increased oestrogen deprivation and efficient launch of inflammatory response. 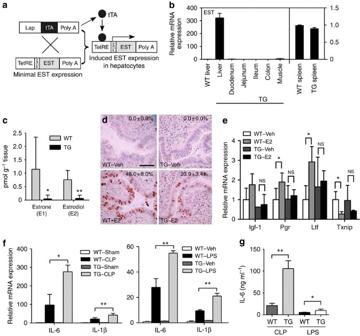Figure 5: TG overexpression of EST in the liver compromised oestrogen activity and sensitized mice to sepsis-responsive inflammatory response. (a) Schematic representation of the Tet-off Lap-tTA/TetRE-EST TG system. (b) Expression of EST in the liver and spleen of WT mice and in different tissues of TG mice as measured by real-time PCR. (c) The hepatic oestrone (E1) and oestradiol (E2) levels were measured in 4-week-old virgin female WT and TG mice. (d) BrdU labelling and immunostaining on uterine paraffin sections from mice of indicated genotype and drug treatment. All mice were ovariectomized 7 days before the oestrogen treatment. Mice received a single subcutaneous injection of vehicle (Veh) or E2(20 μg kg−1) 20 h before being killed. Mice were labelled with BrdU (60 mg kg−1) 2 h before being killed. Percentages of BrdU-positive nuclei are quantitated and labelled. Scale bar, 50 μm. (e) Expression of uterine oestrogen-responsive genes as measured by real-time PCR. (f) CLP- and LPS-responsive expression of inflammatory cytokines in female WT and TG mice. (g) Serum IL-6 level in WT and TG mice subjected to CLP or LPS treatment. The WT and TG groups inc–gcontained four and five independent mice per group, respectively. The mRNA expression levels in the control groups inb,eandfwere arbitrarily set at 1. Results are presented as means±s.d. *P<0.05; **P<0.01; NS, statistically not significant. Student’st-test was used to calculate thePvalues. Igf-1, insulin-like growth factor 1; Ltf, lactoferrin; Pgr, progesterone receptor; Txnip, thioredoxin-interacting protein. Figure 5: TG overexpression of EST in the liver compromised oestrogen activity and sensitized mice to sepsis-responsive inflammatory response. ( a ) Schematic representation of the Tet-off Lap-tTA/TetRE-EST TG system. ( b ) Expression of EST in the liver and spleen of WT mice and in different tissues of TG mice as measured by real-time PCR. ( c ) The hepatic oestrone (E 1 ) and oestradiol (E 2 ) levels were measured in 4-week-old virgin female WT and TG mice. ( d ) BrdU labelling and immunostaining on uterine paraffin sections from mice of indicated genotype and drug treatment. All mice were ovariectomized 7 days before the oestrogen treatment. Mice received a single subcutaneous injection of vehicle (Veh) or E 2 (20 μg kg −1 ) 20 h before being killed. Mice were labelled with BrdU (60 mg kg −1 ) 2 h before being killed. Percentages of BrdU-positive nuclei are quantitated and labelled. Scale bar, 50 μm. ( e ) Expression of uterine oestrogen-responsive genes as measured by real-time PCR. ( f ) CLP- and LPS-responsive expression of inflammatory cytokines in female WT and TG mice. ( g ) Serum IL-6 level in WT and TG mice subjected to CLP or LPS treatment. The WT and TG groups in c – g contained four and five independent mice per group, respectively. The mRNA expression levels in the control groups in b , e and f were arbitrarily set at 1. Results are presented as means±s.d. * P <0.05; ** P <0.01; NS, statistically not significant. Student’s t -test was used to calculate the P values. Igf-1, insulin-like growth factor 1; Ltf, lactoferrin; Pgr, progesterone receptor; Txnip, thioredoxin-interacting protein. Full size image The current study revealed an unexpected role of EST in sepsis response. Sepsis induced hepatic EST gene expression and compromised oestrogenic activity in the liver. Reciprocally, the expression and regulation of EST affected the host’s sensitivity to sepsis. EST ablation and overexpression attenuated and enhanced sepsis-responsive inflammatory response, respectively. The heightened CLP-induced death in EST−/− mice, although paradoxical, was consistent with previous reports that oestrogen receptor agonists increase mortality in endotoxaemic mice [12] , [13] , [14] , [15] . Our results were also consistent with a clinical report that higher oestrogen levels were associated with a greater risk of mortality in critically injured adults [29] . In primary Kupffer cells, in addition to the induction of EST by LPS, we found the lipopeptide Pam3CSK4 was effective, whereas the CpG oligonucleotide ODN1826 was not effective in inducing the EST gene expression. Lipopeptide and CpG oligonucleotide are ligands for TLR2 and TLR9, respectively [16] , [17] . These results suggested that the induction of EST in Kupffer cells was bacterial component dependent and/or TLR isoform dependent. The CLP-sensitizing effect of EST ablation was recapitulated in WT mice treated with the EST inhibitor triclosan. Triclosan is widely used in consumer products as an antibacterial agent, although its antibacterial benefit has recently been questioned. Triclosan inhibits EST from transferring a sulfuryl moiety from the sulfate donor 3′-phosphoadenosine 5′-phosphosulfate onto oestrogen by binding to the oestrogen-binding site on EST, causing the formation of triclosan–sulfate conjugate instead of the oestrogen–sulfate conjugate [23] , [24] . Our results urge caution in avoiding unwanted side effect when the EST-inhibiting pharmaceutical or neutraceutical agents are used in patients of sepsis. The sepsis induction of EST and the establishment of EST as a NF-κB-target gene were surprises considering that many of the drug-metabolizing enzymes are suppressed by inflammation and NF-κB (ref. 11 ). To our knowledge, EST is the first drug-metabolizing enzyme whose expression was reported to be induced by inflammation. The inflammatory responsive induction of EST may represent a double-edged sword. Although the consequent increase in oestrogen deprivation has a potential to exacerbate inflammation as suggested by the results from our EST TG mice, the inflammation sensitizing effect of EST has a potential benefit in helping with the host’s ability to launch an efficient inflammatory response, a key survival response to release pro-inflammatory cytokines and chemokines with subsequent recruitment of inflammatory cells [25] . Inflammation is also associated with many other diseases, including the sterile inflammation seen in various liver diseases, such as the drug-induced liver injury, non-alcoholic and alcoholic steatohepatitis, and liver ischaemia and reperfusion [30] . It is interesting to know whether sterile inflammation, such as that caused by the liver ischaemia and reperfusion, can also induce EST and impact the ischaemia and reperfusion responses. Future studies are also necessary to determine whether a chronic inflammation will result in a sustained induction of EST and if so, what will be the pathophysiological relevance and consequence of a sustained EST induction. The reciprocal regulation of inflammation and EST represents a yet-to-be-explored mechanism of endocrine regulation of inflammation, which may be explored to improve the clinical management of sepsis. Animals and LPS treatment The Tet-off EST TG system is composed of two transgenes, TetRE-EST and Lap-tTA . The creation of the TetRE-EST transgenic line was previously reported by us [31] . The liver-specific Lap-tTA transgenic line was obtained from the Jackson Laboratories (Bar Harbor, ME). Driven by the Lap gene promoter, the Lap-tTA targets the expression of tTA specifically to the hepatocytes [32] . The TetRE-EST/Lap-tTA bitransgenic mice were generated by crossbreeding. Transgenic mice and their wide-type littermates used in this study were maintained in C57BL/6J background. The EST−/− mice [4] and the global TLR4−/− mice [19] have been previously described. C3H/HeJ mice and C3H/HeOuJ mice were purchased from the Jackson Laboratories. LPS was dissolved in PBS and given by intraperitoneal (i.p.) injection. When necessary, mice were pretreated with 200 mg kg −1 PDTC by i.p. injection 1 h before challenging with 5 mg per kg LPS. The majority of the experiments were performed on mice of 8 weeks of age except those specified for ovariectomy (5 week old) and measurement of LPS effect on circulating oestrogen levels (4 week old). All mice used were females except those used in Fig. 4g . All mice used were 6–8 weeks old except those used for ovariectomy and measurement of circulating estrogens as described above. The use of mice in this study has complied with all relevant federal guidelines and institutional policies, and was approved by the University of Pittsburgh Institutional Animal Care and Use Committee. Measurement of uterine oestrogen response Five-week-old virgin females were subjected to ovariectomies. Mice were given a single subcutaneous injection of E 2 (20 μg kg −1 ) 7 days after the surgery. Mice were given a single i.p. injection of bromodeoxyuridine (BrdU, 60 mg kg −1 ) 18 h after the E 2 injection and killed after 2 h. One uterine horn was collected for paraffin section and BrdU immunostaining, and the other was collected for RNA extraction and gene expression analysis by real-time PCR. When necessary, mice were given an i.p. injection of LPS (5 mg kg −1 ) 12 h before the E 2 treatment. Oestrogen sulfotransferase activity assay Liver cytosols were prepared by homogenizing tissues in 5 mmol l −1 KPO 4 buffer (pH 6.5) containing 0.25 mol l −1 sucrose. The cytosols were then used for sulfotransferase assay by using [ 35 S]-phosphoadenosine phosphosulfate from Perkin-Elmer (Waltham, MA) as the sulfate donor [6] . In brief, 20 μg ml −1 total liver cytosolic extract was incubated with 1 μM of oestrone substrate at 37 °C for 30 min. The reaction was terminated by adding ethyl acetate, and the aqueous phase was then counted in the Beckman LS6500 scintillation counter. Measurement of serum and liver tissue oestrogen levels The serum concentrations of oestradiol (E 2 ) were measured using the Ultra-Sensitive Estradiol RIA kit (DSL-4800) from Beckman Coulter (Brea, CA). The liver tissue levels of oestrone (E 1 ) and E 2 were measured by a Ultra performance liquid chromatography tandem mass spectrometry (UPLC/MS–MS) method with a Waters Acquity UPLC system connected with the Xevo TQ triple quadrupole mass spectrometer as we have previously described [33] , [34] . In brief, a Xevo TQ triple quadruple mass spectrometer (Waters, Milford, MA, USA) recorded MS and MS/MS spectra using electrospray ionization in positive-ion and negative-ion modes, capillary voltage of 3.0 kV, extractor cone voltage of 3 V and detector voltage of 650 V. Cone gas flow was set at 50 l h −1 , and desolvation gas flow was maintained at 600 l h −1 . Source temperature and desolvation temperatures were set at 150 and 350 °C, respectively. Analytical separations were conducted on the UPLC system using an Acquity UPLC HSS T3 1.8 μm 1 × 150 mm analytical column kept at 50 °C and at a flow rate of 0.15 ml min −1 . Kupffer cell isolation and drug treatment The mouse primary Kupffer cells were isolated as described by others [35] . Briefly, the mouse liver was digested by collagenase perfusion. After removing the undigested tissue, the cell suspension was processed with gradient centrifugation to isolate Kupffer cells. After 2 h of culture, the non-adherent cells were removed and the remaining adherent cells were further cultured as Kupffer cells. When necessary, Kupffer cells were treated with LPS (1 μg ml −1 ), Pam3CSK4 (300 ng ml −1 ) or ODN1826 (10 μg ml −1 ) for 16 h before RNA collection and real-time PCR analysis. Pam3CSK4, ODN1826 and the control ODN were purchased from InvivoGen (San Diego, CA). Real-time PCR analysis Total RNA was extracted from tissues using the TRIzol reagent from Invitrogen. Reverse transcription was performed with iScript cDNA Synthesis Kit from Bio-Rad (Hercules, CA). SYBR Green-based real-time PCR was performed with the ABI 7300 Real-Time PCR System. Data were normalized against the control of cyclophilin signals. The mRNA expression levels in the control groups were arbitrarily set at 1. The sequences of the PCR primers are listed in Supplementary Table 1 . Western blot analysis Mouse liver tissue was homogenized in radioimmunoprecipitation assay lysis buffer (50 mM Tris (pH 8.0), 150 mM sodium chloride, 1.0%Triton X-100, 0.5% sodium deoxycholate, 0.1% SDS). The protein concentrations in the supernatants were quantified, and 50 μg total proteins for each sample was separated on 10% SDS–polyacrylamide gel and transferred to a polyvinylidenedifluoride membrane. The membrane was blocked with 5% milk in 1 × Tris-Buffered Saline and Tween 20 (TBST) buffer followed by overnight incubation at 4 °C with primary polyclonal rabbit antibody against EST/SULT1E1 (Cat # 12522-1-AP; 1:500) from Proteintech (Chicago, IL) and then with a secondary antibody for 1 h at room temperature. After washing the membrane with 1 × TBST, the membrane was incubated with chemiluminescent substrate and exposed against the Kodak X-ray film. Monoclonal mouse antibody against β-actin (1:5,000) was used as a loading control. The original Western blots are shown in Supplementary Figure 5 . Caecal ligation and puncture model This was performed essentially as described [1] . In brief, mice were anesthetized with a mixture of ketamine (150 mg kg −1 ) and xylazine (10 mg kg −1 ) by i.p. injection. Under aseptic conditions, a 2-cm midline laparotomy was performed to allow the exposure of the caecum with the adjoining intestine. The caecum was 50% ligated with a 4.0 silk suture at its base, below the ileocaecal valve, and was perforated twice with an 18-gauge needle (top and bottom). Twenty-one gauge needles were used in CLP survival experiments when the TG mice were used to avoid excessive injury. The caecum was then gently squeezed to extrude a small amount of faeces from the perforation sites. The caecum was then returned to the peritoneal cavity and the laparotomy was closed with 4.0 silk sutures. The fluid resuscitation was provided after CLP as described [1] . All mice were then returned to their home cages with free access to food and water, and killed 12 h after the surgery. When necessary, mice were given daily subcutaneous injections of triclosan (10 mg kg −1 , Cat #72779 from Sigma) beginning 3 days before CLP. Also when necessary, mice were pretreated with PDTC (200 mg kg −1 ) by i.p. injection 1 h before CLP, or CLP was performed 7 days after ovariectomy. The bacterial count in the peritoneal fluid was measured as we have previously described [2] . In brief, the peritoneal cavity was washed with 1 ml PBS, and the peritoneal lavage was collected under sterile conditions. Peritoneal lavage fluid was subjected to serial 10-fold dilutions and cultured overnight in 5% sheep blood agar (Teknova, Hollister, CA). Colony-forming unit was quantified by manual counting. Kupffer cell depletion Eight-week-old mice were treated with saline or 20 mg per kg gadolinium chloride (GdCl 3 , 2 mg ml −1 ) from Sigma-Aldrich via tail vein injection. Twenty-four hours later, mice were again given the same dose of GdCl 3 before being treated with 5 mg kg −1 of LPS by i.p. injection or subjected to CLP. Mice were killed 12 h after LPS or CLP treatment. Cell culture and transfection and reporter gene assay HepG2 cells were maintained in Dulbecco’s modified Eagle medium supplemented with 10% fetal bovine serum. The 2.5- and 1.5-kb 5′-regulatory sequences of the mouse EST gene were amplified by PCR using mouse genomic DNA as the template and subsequently cloned into the pGL3-basic vector from Clontech (Mountain View, CA). The mutant promoter reporter genes were generated by PCR-mediated mutagenesis. HepG2 cells were transiently transfected with the reporter constructs and the p65 expression vector (pCMV-p65) in 48-well plates by using the polyethylenimine polymer transfection agent [36] . Cells were then collected and measured for luciferase and β-gal activities 24 h after transfection. Transfection efficiency was normalized against β-gal activity derived from the co-transfected pCMX–β-gal plasmid. All EST promoter activities were normalized to EST 2.5-kb vector, which was arbitrarily set at 1. EMSA and ChIP assay The p65 protein was synthesized using the T7 Quick Coupled Transcription/Translation System in vitro transcription and translation system from Promega (Madison, WI). EMSA was performed by using 32 P-labelled oligonucleotides and p65 protein [6] . In the ChIP assay, 4-week-old WT female mice received a single i.p. injection of LPS (5 mg kg −1 ) 12 h before liver collection. The ChIP assay was performed as we have previously described [36] . In brief, liver tissue lysates were incubated overnight with an anti-p65 antibody (Clone L8F6, Cat # 6956) from Cell Signaling (Danvers, MA) at 4 °C. The precipitated complexes were collected with protein A–agarose/salmon sperm DNA. DNA in the precipitated samples were reverse cross-linked at 65 °C for 4 h and the DNA were recovered by phenol/chloroform extraction and ethanol precipitation before subjecting to real-time PCR analysis. In the ChIP assay, the recruitment of p65 in the vehicle group was arbitrarily set at 1. The original EMSA blots are shown in Supplementary Figure 6 . Statistical analysis When applicable, results are presented as means±s.d. Statistical analysis was performed using the student’s t -test for comparison between two groups. The Log-rank (Mantel–Cox) test was used to compare the survival profiles. P values of <0.05 were considered statistically significant. How to cite this article: Chai, X. et al. Oestrogen sulfotransferase ablation sensitizes mice to sepsis. Nat. Commun. 6:7979 doi: 10.1038/ncomms8979 (2015).